A glutamatergic reward input from the dorsal raphe to ventral tegmental area dopamine neurons Electrical stimulation of the dorsal raphe (DR) and ventral tegmental area (VTA) activates the fibres of the same reward pathway but the phenotype of this pathway and the direction of the reward-relevant fibres have not been determined. Here we report rewarding effects following activation of a DR-originating pathway consisting of vesicular glutamate transporter 3 (VGluT3) containing neurons that form asymmetric synapses onto VTA dopamine neurons that project to nucleus accumbens. Optogenetic VTA activation of this projection elicits AMPA-mediated synaptic excitatory currents in VTA mesoaccumbens dopaminergic neurons and causes dopamine release in nucleus accumbens. Activation also reinforces instrumental behaviour and establishes conditioned place preferences. These findings indicate that the DR–VGluT3 pathway to VTA utilizes glutamate as a neurotransmitter and is a substrate linking the DR—one of the most sensitive reward sites in the brain—to VTA dopaminergic neurons. Electrical stimulation of the brain has been useful in the identification of many brain sites thought to have roles in reward. Two particularly interesting sites are the dorsal raphe (DR), where stimulation produces reward-relevant responding at among the highest rates and lowest thresholds [1] and the ventral tegmental area (VTA), the origin of dopamine pathways implicated in reward function by pharmacological studies [2] . That the two sites are connected by common reward-associated fibres has been established by dual-electrode, paired-pulse stimulation experiments [3] , but these experiments reveal neither the origin nor the target of the activated substrate. Although the DR is best known as the origin of a multi-branching serotonergic pathway that projects to VTA, DR neurons that express VGluT3 also project to the VTA [4] and offer a potential substrate for reward-related function. That glutamate is likely to be the neurotransmitter of reward-related afferents to dopaminergic (DA) neurons is suggested by the fact that DA neurons respond to reward signals by burst firing [5] , and that burst firing by DA neurons is a response to glutamatergic inputs [6] . In the present study we identified a glutamatergic pathway that carries reward signals from the DR to the VTA DA system. Using anatomical and optogenetic approaches, we found that the major subpopulation of DR neurons projecting to the VTA expresses VGluT3 in the rat and in the mouse, and within the VTA, axon terminals from DR–VGluT3 neurons form asymmetric synapses mostly on DA neurons. At least some of the DA neurons targeted by DR–VGluT3 inputs innervate the nucleus accumbens (nAcc), and light stimulation of this DR–VGluT3 pathway to VTA elicits AMPA-mediated excitatory currents in VTA-DA neurons, promotes DA release in nAcc, reinforces instrumental behaviour, and establishes conditioned place preference. We propose this glutamatergic pathway as the first fully characterized synaptic link between electrically stimulated reward circuitry within the DR and the dopamine system on which it depends. Most rat DR neurons innervating the VTA express VGluT3 mRNA VGluT3 neurons and serotonergic neurons from DR are known to innervate the rat VTA [4] , [7] , [8] , [9] , [10] , [11] . To determine the relative proportions of rat DR neurons projecting to VTA expressing VGluT3, the rate-limiting enzyme for serotonin production (tryptophan hydroxylase; TPH), or both markers, we first injected the retrograde tracer Fluoro-Gold (FG) into the rat VTA ( Fig. 1a,b and Supplementary Fig. 1 ). We then looked for co-localization of FG ( Fig. 1c,d ) with VGluT3 mRNA, using in situ hybridization ( Fig. 1e ), or TPH, using immunohistochemistry ( Fig. 1f ). We found that about half of all FG neurons expressed VGluT3 mRNA without TPH (45.54±1.24%; 1,329 cells out of 2,968 FG neurons; Fig. 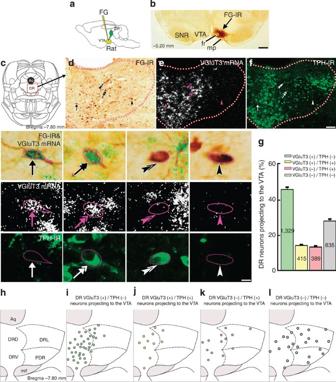Figure 1: Most DR neurons projecting to the VTA express VGluT3 mRNA. (a) Retrograde tracer FG was delivered into the VTA. (b) FG injection site in the VTA. (c) DR diagram. (d–f) Low magnification of a DR coronal section showing brown cells with FG-immunoreactivity (FG-IR,d), expression of VGluT3 mRNA (white aggregated grains;e) or TPH-immunoreactivity (TPH-IR, green;f). Four individual cells are seen at higher magnification. A FG neuron expressing VGluT3 mRNA without TPH-IR (arrow), a FG neuron co-expressing VGluT3 mRNA and TPH-IR (double arrow), a FG neuron expressing TPH-IR only (double arrowheads) and a FG neuron lacking both VGluT3 mRNA and TPH-IR (arrowhead). (g) Frequency of FG phenotypes (mean+s.e.m.). Among all DR neurons projecting to the VTA, 46% expressed only VGluT3 mRNA, 14% co-expressed VGluT3 mRNA and TPH-IR, 13% expressed TPH-IR alone and 28% lacked both VGluT3 mRNA and TPH-IR. FG cell counting was made between bregma −6.84 and −8.40 mm (n=4, 10–15 sections per rat). (h–l) Phenotype map of DR neurons projecting to the VTA. Each dot represents the average of DR neurons projecting to the VTA. Many VGluT3 expressing neurons without TPH-IR were concentrated in the dorsal part (DRD) and ventral part (DRV) of the DR (green;i) intermixed with neurons that either co-expressed TPH-IR with VGluT3 (yellow;j) or expressed only TPH-IR (pink;k). DR neurons projecting to the VTA lacking both VGluT3 and TPH-IR were frequently observed in the DRD, DRV, lateral (DRL) and posterodorsal (PDR) aspects of the DR (grey;l). Aq, aqueduct; fr, fasciculus retroflexus; mlf, medial longitudinal fasciculus; mp, mammillary peduncle; SNR, substantia nigra reticulata. Diagrams were adapted from rat brain atlas57. Bars, (b) 400 μm; (f) 110 μm; 10 μm for high magnification. 1g and Supplementary Table 1 ). Some FG neurons co-expressed VGluT3 mRNA and TPH (13.99±0.81%; 415 cells out of 2,968 FG neurons), whereas others expressed TPH without VGluT3 mRNA (12.90±0.91%; 389 cells out of 2,968 FG neurons). A fourth subpopulation of FG neurons lacked both VGluT3 mRNA and TPH (27.65±1.36%; 835 cells out of 2,968 FG neurons). Most of the FG neurons expressing VGluT3 without TPH were concentrated in the dorsal and ventral aspects of the DR ( Fig. 1h,i ), and were intermingled with FG-TPH neurons co-expressing ( Fig. 1j ) or lacking VGluT3 ( Fig. 1k ). The FG neurons lacking both VGluT3 and TPH were observed in all aspects of the DR ( Fig. 1l ). Although it is well documented that the VTA receives a major serotonergic input from the DR [7] , [8] , [9] , [10] , our findings indicate that the major projection from rat DR to VTA consists of VGluT3 neurons (58.76%), with a minor pathway arising from a population of TPH neurons without VGluT3 (12.90%). Although most of the DR VGluT3 neurons projecting to the VTA lacked TPH, nearly half of all TPH neurons co-expressed VGluT3 mRNA (51.61%). These data suggest that the majority of inputs from the DR to the VTA have the capacity to accumulate glutamate into synaptic vesicles via VGluT3. Figure 1: Most DR neurons projecting to the VTA express VGluT3 mRNA. ( a ) Retrograde tracer FG was delivered into the VTA. ( b ) FG injection site in the VTA. ( c ) DR diagram. ( d – f ) Low magnification of a DR coronal section showing brown cells with FG-immunoreactivity (FG-IR, d ), expression of VGluT3 mRNA (white aggregated grains; e ) or TPH-immunoreactivity (TPH-IR, green; f ). Four individual cells are seen at higher magnification. A FG neuron expressing VGluT3 mRNA without TPH-IR (arrow), a FG neuron co-expressing VGluT3 mRNA and TPH-IR (double arrow), a FG neuron expressing TPH-IR only (double arrowheads) and a FG neuron lacking both VGluT3 mRNA and TPH-IR (arrowhead). ( g ) Frequency of FG phenotypes (mean+s.e.m.). Among all DR neurons projecting to the VTA, 46% expressed only VGluT3 mRNA, 14% co-expressed VGluT3 mRNA and TPH-IR, 13% expressed TPH-IR alone and 28% lacked both VGluT3 mRNA and TPH-IR. FG cell counting was made between bregma −6.84 and −8.40 mm ( n =4, 10–15 sections per rat). ( h – l ) Phenotype map of DR neurons projecting to the VTA. Each dot represents the average of DR neurons projecting to the VTA. Many VGluT3 expressing neurons without TPH-IR were concentrated in the dorsal part (DRD) and ventral part (DRV) of the DR (green; i ) intermixed with neurons that either co-expressed TPH-IR with VGluT3 (yellow; j ) or expressed only TPH-IR (pink; k ). DR neurons projecting to the VTA lacking both VGluT3 and TPH-IR were frequently observed in the DRD, DRV, lateral (DRL) and posterodorsal (PDR) aspects of the DR (grey; l ). Aq, aqueduct; fr, fasciculus retroflexus; mlf, medial longitudinal fasciculus; mp, mammillary peduncle; SNR, substantia nigra reticulata. Diagrams were adapted from rat brain atlas [57] . Bars, ( b ) 400 μm; ( f ) 110 μm; 10 μm for high magnification. Full size image Most DR-VGluT3 axons synapse on TH-positive dendrites A prior study using pressure injections and non-radioactive detection of VGluT3 mRNA reported that all VGluT3 afferents to VTA were from the DR and the bed nucleus of the stria terminalis [4] . In the present study by using iontophorectic application of FG (to minimize labelling of fibres of passage) and radioactive detection of VGluT3 mRNA (to maximize detection of mRNA), we confirmed that DR VGluT3 neurons project to the VTA, and found very few VGluT3 neurons from the medial raphe projecting to the VTA, but did not find VGluT3 neurons from the bed nucleus of the stria terminalis projecting to the VTA ( Supplementary Fig. 2 ). These findings together with prior studies showing lack of VGluT3 mRNA in the VTA [12] , [13] suggest that the major source of VGluT3 afferents, if not the only one, to the VTA is from the DR. To determine whether DR VGluT3 terminals form synapses on VTA tyrosine hydroxylase (TH) neurons, we performed double VGluT3 and TH immuno-electron microscopy with an anti-VGluT3 antibody that in the DR labelled only those neurons that co-expressed VGluT3 mRNA ( Supplementary Fig. 3 ). By using this anti-VGluT3 antibody, we found that VGluT3-terminals established asymmetric synapses mostly on TH-positive dendrites (62.51±0.44%; 291 terminals out of 466; Fig. 2a,c ), and less frequently on TH-negative dendrites (37.49±0.44%; 175 terminals out of 466; Fig. 2b,c ). The presence of VGluT3-axon terminals making asymmetric synapses in the VTA suggests that these terminals provide an excitatory input to VTA neurons. Thus, we next examined whether glutamatergic receptors were found postsynaptic to VGluT3 terminals. By fluorescence microscopy, we detected in the VTA the AMPA receptor subunit GluR1 postsynaptic to VGluT3 punctuate structures that were distributed within TH-positive neurons ( Fig. 2d,e ). By immuno-electron microscopy, we confirmed the presence of GluR1 along the postsynaptic membrane of asymmetric synapses established by VGluT3 axon terminals ( Fig. 2f ). These anatomical findings indicate that the DR provides a major glutamatergic input to TH neurons in the VTA. 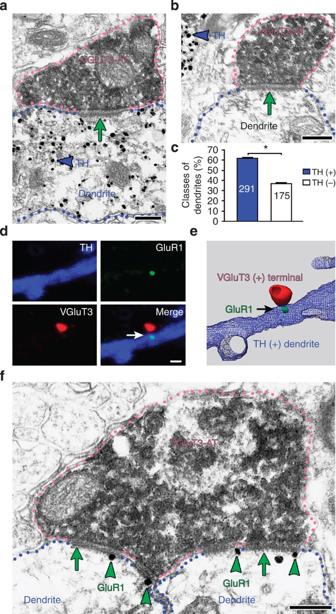Figure 2: VGluT3 neurons make asymmetric synapses on TH neurons having GluR1 postsynaptic to VGluT3 terminals. (a–c) VGluT3 terminals make synapses mostly on TH-positive dendrites (electron microscopy). (a) An axon terminal (AT) containing VGluT3 (scattered dark material) makes an asymmetric synapse (green arrow) with a TH-positive (gold particles, blue arrowhead) dendrite. (b) An axon terminal containing VGluT3 makes an asymmetric synapse (green arrow) with a TH-negative dendrite. (c) The bars indicate the frequency (mean+s.e.m.) of VGluT3 terminals making asymmetric synapses on TH-positive or TH-negative dendrites. From a total of 466 VGluT3 terminals, 62.51±0.44% (n=291) make synapses on TH-positive dendrites and 37.49±0.44% (n=175) on TH-negative dendrites (*P<0.0001,t3=28.65, two-tailed pairedt-test, terminals collected from four rats,n=number of counted terminals). (d) A TH-positive dendrite containing GluR1 signal postsynaptic to a VGluT3 terminal (immunofluorescence microscopy). Note the presence of GluR1 (green, arrow) located within a TH-positive dendrite (blue) adjacent to a VGluT3-positive terminal (red). (e) The association between the postsynaptic GluR1 within a TH dendrite and a VGluT3 terminal is better seen after three-dimensional reconstruction of confocal images. (f) At the electron microscopic level, GluR1 signal is seen as gold particles (arrowheads) along the postsynaptic membrane of two dendrites making asymmetric synapses (arrows) with a single AT (pink outline) containing VGluT3 (scattered dark material). Bars, (a,bandf) 200 nm; (d) 2 μm. Figure 2: VGluT3 neurons make asymmetric synapses on TH neurons having GluR1 postsynaptic to VGluT3 terminals. ( a – c ) VGluT3 terminals make synapses mostly on TH-positive dendrites (electron microscopy). ( a ) An axon terminal (AT) containing VGluT3 (scattered dark material) makes an asymmetric synapse (green arrow) with a TH-positive (gold particles, blue arrowhead) dendrite. ( b ) An axon terminal containing VGluT3 makes an asymmetric synapse (green arrow) with a TH-negative dendrite. ( c ) The bars indicate the frequency (mean+s.e.m.) of VGluT3 terminals making asymmetric synapses on TH-positive or TH-negative dendrites. From a total of 466 VGluT3 terminals, 62.51±0.44% ( n =291) make synapses on TH-positive dendrites and 37.49±0.44% ( n =175) on TH-negative dendrites (* P <0.0001, t 3 =28.65, two-tailed paired t -test, terminals collected from four rats, n =number of counted terminals). ( d ) A TH-positive dendrite containing GluR1 signal postsynaptic to a VGluT3 terminal (immunofluorescence microscopy). Note the presence of GluR1 (green, arrow) located within a TH-positive dendrite (blue) adjacent to a VGluT3-positive terminal (red). ( e ) The association between the postsynaptic GluR1 within a TH dendrite and a VGluT3 terminal is better seen after three-dimensional reconstruction of confocal images. ( f ) At the electron microscopic level, GluR1 signal is seen as gold particles (arrowheads) along the postsynaptic membrane of two dendrites making asymmetric synapses (arrows) with a single AT (pink outline) containing VGluT3 (scattered dark material). Bars, ( a , b and f ) 200 nm; ( d ) 2 μm. Full size image DR VGluT3 neurons synapse on mesoaccumbens TH neurons We next characterized the mouse DR–VTA pathway ( Supplementary Fig. 4 ), and determined that as in the rat, most of the mouse DR neurons projecting to the VTA had VGluT3 (67%; Supplementary Fig. 5 ). After validating similarities between rat and mouse DR–VTA projections, we selectively labelled the mouse VGluT3 terminals from DR to the VTA by injecting the adeno-associated virus encoding Cre-dependent ChR2 tethered to mCherry into the DR of mice expressing Cre-recombinase under the regulation of the VGluT3 promoter (VGluT3-ChR2-mCherry mice; Fig. 3a ). By DR dual immunofluorescence, we confirmed the expression of VGluT3 in almost all mCherry neurons (98.52±0.001%; 1,596 VGluT3-mCherry neurons out of 1,619 mCherry neurons; 24 sections from four VGluT3-ChR2-mCherry mice, Supplementary Fig. 6 ). These findings indicate the selective expression of mCherry under the VGluT3 promoter. To determine whether mouse VGluT3 neurons targeted VTA TH-neurons innervating the nAcc, the mesoaccumbens neurons were labelled by injection of FG into the mouse nAcc, and VTA synapses were examined ( Fig. 3a,b ). By triple immunofluorescence, we found that VGluT3 inputs from the DR targeted TH dendrites containing FG signal ( Fig. 3c–f ). By electron microscopic analysis of triple-immunolabelled VTA, we found that DR VGluT3 axon terminals containing mCherry formed asymmetric synapses on FG-positive mesoaccumbens neurons ( Fig. 3g ). Together these fluorescence and ultrastructural findings indicate that DA mesoaccumbens neurons are targeted by glutamatergic inputs from the DR. 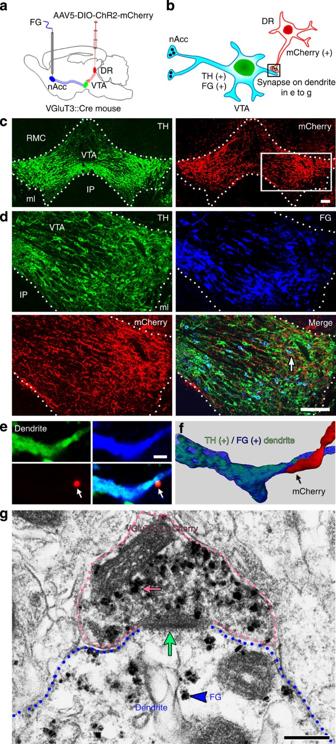Figure 3: VGluT3 axon terminals from DR make asymmetric synapses on VTA dopamine neurons that innervate the nAcc. (a) DR VGluT3 neurons were infected by injections of AAV5-DIO-ChR2-mCherry into the DR of VGluT3::Cre mice (n=3). The retrograde tracer FG was injected into the nAcc to label individual mesoaccumbens neurons. (b) Schematic representation of a mesoaccumbens DA neuron (containing FG) forming an asymmetric synapse with a VGluT3 AT (containing mCherry) from DR. (c–f) VGluT3 inputs from DR target mesoaccumbens DA neurons (immunofluorescence microscopy; TH (green), FG (blue) and mCherry (red)). (d) Delimited area by white box inbis seen at high magnification showing detection of TH, FG and mCherry within the lateral VTA. White arrow pointed to a mesoaccumbens TH neuron, a dendrite from this neuron is shown at higher magnification ine. This TH-FG dendrite is in association with a VGluT3 terminal (from DR) containing mCherry (white arrows). (f) The association between the mesoaccumbens TH dendrite and VGluT3 terminal (arrow) is better seen after three-dimensional reconstruction of confocal images. Bregma at −3.52 mm. RMC, red nucleus magnocellular part; IP, interpeduncular nucleus; ml, medial lemniscus. (g) ATs from DR containing VGluT3 and mCherry make asymmetric synapses on mesoaccumbens neurons (electron microscopy, triple immunolabeling). VGluT3- (gold particles, pink arrow) and FG- (gold particles, blue arrowhead) immunogold labelling combined with mCherry-immunoperoxidase labelling (scattered dark material). An AT (pink outline) co-expressing VGluT3 and mCherry makes an asymmetric synapse (green arrow) with a FG-positive mesoaccumbens dendrite. Bars, (candd) 100 μm; (e) 2 μm; (g) 200 nm. Figure 3: VGluT3 axon terminals from DR make asymmetric synapses on VTA dopamine neurons that innervate the nAcc. ( a ) DR VGluT3 neurons were infected by injections of AAV5-DIO-ChR2-mCherry into the DR of VGluT3::Cre mice ( n =3). The retrograde tracer FG was injected into the nAcc to label individual mesoaccumbens neurons. ( b ) Schematic representation of a mesoaccumbens DA neuron (containing FG) forming an asymmetric synapse with a VGluT3 AT (containing mCherry) from DR. ( c – f ) VGluT3 inputs from DR target mesoaccumbens DA neurons (immunofluorescence microscopy; TH (green), FG (blue) and mCherry (red)). ( d ) Delimited area by white box in b is seen at high magnification showing detection of TH, FG and mCherry within the lateral VTA. White arrow pointed to a mesoaccumbens TH neuron, a dendrite from this neuron is shown at higher magnification in e . This TH-FG dendrite is in association with a VGluT3 terminal (from DR) containing mCherry (white arrows). ( f ) The association between the mesoaccumbens TH dendrite and VGluT3 terminal (arrow) is better seen after three-dimensional reconstruction of confocal images. Bregma at −3.52 mm. RMC, red nucleus magnocellular part; IP, interpeduncular nucleus; ml, medial lemniscus. ( g ) ATs from DR containing VGluT3 and mCherry make asymmetric synapses on mesoaccumbens neurons (electron microscopy, triple immunolabeling). VGluT3- (gold particles, pink arrow) and FG- (gold particles, blue arrowhead) immunogold labelling combined with mCherry-immunoperoxidase labelling (scattered dark material). An AT (pink outline) co-expressing VGluT3 and mCherry makes an asymmetric synapse (green arrow) with a FG-positive mesoaccumbens dendrite. Bars, ( c and d ) 100 μm; ( e ) 2 μm; ( g ) 200 nm. Full size image Mesoaccumbens TH neuronal activation by DR-VGluT3 afferent VGluT3 belongs to a family of three vesicular glutamate transporters (VGluT1, VGluT2 and VGluT3). While VGluT1 and VGluT2 are restricted to known glutamatergic neurons, VGluT3 is found in hippocampal GABAergic neurons, striatal cholinergic interneurons, monoamine neurons and glia [14] , [15] , [16] . To determine the capacity of DR VGluT3 efferents to release glutamate on mesoaccumbens neurons, intracellular recordings were performed in VTA slices from VGluT3-ChR2-eYFP mice injected in the nAcc with the retrograde tract tracer Dil ( n =6; Fig. 4a and Supplementary Fig. 7a,b ). A total of 37 DiI-labelled VTA neurons were recorded, and were classified into two subpopulations on the basis of action potential width during cell attached recordings, and peak firing frequency in response to depolarizing current ( Supplementary Fig. 7 ). Light-activated excitatory postsynaptic currents (EPSCs) were observed in nearly one-half of the Dil-labelled neurons (18/37; Supplementary Fig. 7 ); consistent with anatomical data demonstrating VGluT3 inputs on mesoaccumbens neurons from the DR nucleus. The majority of the neurons (type 1; n =13) exhibited long-duration action potentials (2.36±0.28 ms) and low-to-moderate firing frequencies during depolarization (6.92±0.71 Hz). Type 1 neurons exhibited large inward ‘sag’ currents during strong membrane hyperpolarization (117.67±30.28 pA at −110 mV), consistent with the activation of hyperpolarization-activated cation ( I h ) currents. The remaining neurons (type 2; n =5) exhibited short-duration action potentials (1.20±0.08 ms), fast firing frequencies during depolarization (95.40±6.94 Hz) and small inward currents during hyperpolarization (46.09±21.24 pA). By immunohistochemistry, we found that type 1 neurons were TH-positive, and type 2 neurons were TH-negative ( Fig. 4b,d and Supplementary Fig. 7 ). TH-positive neurons showed larger mean light-evoked EPSCs (−37.53±11.71 pA) using maximal stimulation parameters (10 mW, 5 ms) than the TH-negative neurons (−9.85±4.45 pA; Supplementary Fig. 7i ). However, there was still considerable heterogeneity within individual TH-positive neurons (range −5 to −133 pA). Input–output curves ( Supplementary Fig. 7 ) and pharmacological manipulations were only performed in TH-positive neurons with reliably detectable, larger responses (≥20 pA). Larger light-activated currents in TH-positive neurons were negatively correlated with the amplitude of the I h currents, although this did not achieve statistical significance ( Fig. 4d,e ; Pearson’s correlation coefficient r =−0.5145, P =0.07). Consistent with the presence of GluR1 at postsynaptic sites, light-evoked currents were blocked by the AMPA/kainate receptor antagonist DNQX ( Fig. 4g ). In current clamp recordings, light-evoked EPSPs elicited in TH-positive neurons were capable of driving action potentials across a range of frequencies ( n =5), and firing was prevented by DNQX application ( Fig. 4g,h ). To further determine the monosynaptic nature of the DR VGluT3-VTA projections, VTA EPSCs evoked by light stimulation of DR inputs were recorded in the presence of tetrodotoxin (TTX; 500 nM). We found that TTX eliminated the optical-evoked EPSCs, which were restored by subsequent application of 4-aminopyridine (200 μM) in the presence of TTX ( Supplementary Fig. 8a–c ). We also observed that the light-evoked EPSCs exhibited short latency (2.08±0.13 ms, n =7) and low synaptic jitter (s.d. of latency) (0.22±0.05 ms, n =7; Supplementary Fig. 8d ). From these electrophysiological findings, we inferred that some mesoaccumbens DA neurons receive monosynaptic glutamatergic signalling from DR-VGluT3 fibres, which are capable of driving mesoaccumbens neuronal firing. In vivo this would be expected to evoke DA release within the nAcc. 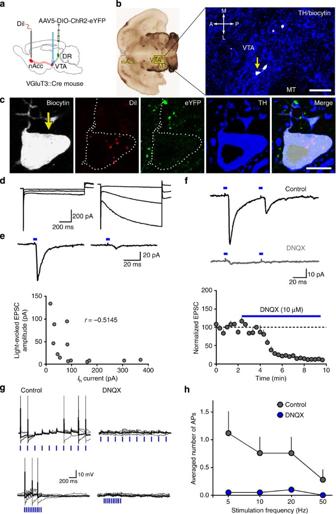Figure 4: Glutamate release onto mesoaccumbens neurons is driven by light-evoked activation of fibres from DR VGluT3 neurons. (a) DR VGluT3 neurons were infected by AAV5-DIO-ChR2-eYFP injected into the DR of VGluT3::Cre mice. The retrograde tracer DiI was injected into the nAcc to label individual mesoaccumbens neurons for intracellular recordings. (b) Brain horizontal section, containing biocytin filled cells (white cells) in VTA (TH immunoreactivity, blue). (c) At higher magnification note a biocytin cell with both DiI (red dots) and TH (blue), and DR VGluT3 terminals containing eYFP (green). (d) Responses of two TH-positive, mesoaccumbens neurons to hyperpolarizing voltage steps (−70, −90 and −110 mV) and (e) light-evoked EPSCs from the same neurons (blue boxes; onset of the laser pulses). Larger light-evoked EPSCs were observed in cells lacking large hyperpolarization-activated currents (Pearson’s correlation coefficientr=−0.5145,P=0.07). (f) Traces from an individual neuron obtained before (control) and during 10 μM DNQX application. DNQX eliminated currents in all tested cells (P<0.001,t3=53.47,n=4, pairedt-test). Individual (grey) and averaged (black) current clamp traces from a single neuron (−55 mV) during light stimulation at 5 Hz (g, upper panel) and 20 Hz (g, lower panel). DNQX eliminated firing elicited by light. (h) Summary of the average number of action potentials observed during light stimulation in a group of TH-positive mesoaccumbens neurons (treatment × frequency:F1,28=15.76,P=0.005,n=5, five trials per cell; two-way ANOVA) before and after DNQX application. Data are presented as mean+s.e.m. Bars, (b) 100 μm; (c) 10 μm. Figure 4: Glutamate release onto mesoaccumbens neurons is driven by light-evoked activation of fibres from DR VGluT3 neurons. ( a ) DR VGluT3 neurons were infected by AAV5-DIO-ChR2-eYFP injected into the DR of VGluT3::Cre mice. The retrograde tracer DiI was injected into the nAcc to label individual mesoaccumbens neurons for intracellular recordings. ( b ) Brain horizontal section, containing biocytin filled cells (white cells) in VTA (TH immunoreactivity, blue). ( c ) At higher magnification note a biocytin cell with both DiI (red dots) and TH (blue), and DR VGluT3 terminals containing eYFP (green). ( d ) Responses of two TH-positive, mesoaccumbens neurons to hyperpolarizing voltage steps (−70, −90 and −110 mV) and ( e ) light-evoked EPSCs from the same neurons (blue boxes; onset of the laser pulses). Larger light-evoked EPSCs were observed in cells lacking large hyperpolarization-activated currents (Pearson’s correlation coefficient r =−0.5145, P =0.07). ( f ) Traces from an individual neuron obtained before (control) and during 10 μM DNQX application. DNQX eliminated currents in all tested cells ( P <0.001, t 3 =53.47, n =4, paired t -test). Individual (grey) and averaged (black) current clamp traces from a single neuron (−55 mV) during light stimulation at 5 Hz ( g , upper panel) and 20 Hz ( g , lower panel). DNQX eliminated firing elicited by light. ( h ) Summary of the average number of action potentials observed during light stimulation in a group of TH-positive mesoaccumbens neurons (treatment × frequency: F 1,28 =15.76, P =0.005, n =5, five trials per cell; two-way ANOVA) before and after DNQX application. Data are presented as mean+s.e.m. Bars, ( b ) 100 μm; ( c ) 10 μm. Full size image DR-VGluT3 afferents to VTA evoke nAcc DA release We next determined whether light activation of the VGluT3 pathway from DR to VTA elicits DA release in nAcc. We evaluated extracellular nAcc DA levels by microdialysis coupled with HPLC- electrochemical detection in freely moving VGluT3-ChR2-eYFP mice during VTA photostimulation of DR VGluT3-ChR2 inputs ( Fig. 5a ). Basal extracellular nAcc DA levels were not significantly different between wild-type mice (0.39±0.01 nM, n =6) and VGluT3::Cre mice (0.37±0.03 nM, n =12). VTA light activation (1 mW, 10 ms pulses at 20 Hz, 3 s on/off for 10 min) of DR VGluT3 inputs in VGluT3-ChR2-eYFP mice significantly enhanced DA levels in nAcc ( P <0.001 versus VGluT3-eYFP control mice, two-way analysis of variance (ANOVA), Fig. 5b ). DA levels returned quickly to baseline after light offset. To determine whether glutamate receptors on VTA DA neurons mediate this effect, 0.2 μl of AMPA receptor antagonist CNQX (1 μg) or NMDA receptor antagonist AP5 (1 μg) were each microinjected into the VTA of VGluT3-ChR2-eYFP mice 10 min before light stimulation. The nAcc DA release induced by VTA light stimulation of VGluT3 inputs was blocked by VTA CNQX, but unaffected by intra-VTA injections of artificial cerebrospinal fluid (ACSF) or AP5 ( Fig. 5c ). These findings confirm that AMPA receptor activation of DA mesoaccumbens neurons by glutamate release from DR VGluT3 inputs enhances DA levels in the nAcc. 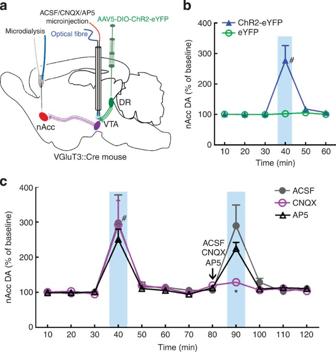Figure 5: Light activation of VTA projections from DR VGluT3 neurons induces nAcc DA release mediated by VTA AMPA receptors. (a) Schematic representation of virus injection in DR of VGluT3::Cre mice, intra-VTA microinjection of AMPA receptor antagonist (CNQX), VTA light stimulation of DR-VGluT3 inputs, and microdialysis in nAcc. (b) VTA light activation of DR VGluT3 inputs induced nAcc DA release. Each point represents a 10-min dialysate sampling period (mean+s.e.m. percent of DA baseline); blue rectangles indicate the period of light stimulation. Light activation significantly enhanced nAcc DA levels in ChR2-eYFP mice (n=6) but not in eYFP mice (n=4) (main effect group: F1,8=96.91,P<0.001; main effect time: F5,40=42.17,P<0.001; group × time interactions: F5,40=40.38,P<0.001, two-way ANOVA). (c) nAcc DA release induced by VTA light activation of DR VGluT3 inputs is abolished by intra-VTA microinjection of CNQX but not AP5. Results were analysed separately for light activation only (10 to 70 min) and light activation following VTA microinjections of ACSF, CNQX or AP5 (80 to 120 min). Light activation significantly enhanced nAcc DA levels in all animals before VTA microinjections (main effect group: F2,15=0.37,P=0.70; main effect time: F6,90=22.36,P<0.001; group × time interactions: F12,90=0.15,P=1.00, two-way ANOVA). The 40-min time point samples were significantly different from all the other time point samples (#P<0.001, Bonferronipost hoctest, ACSF group: 297.7±79.7%,n=6; CNQX group: 292.5±69.3%,n=6; AP5 group: 250.9±29.2%,n=6). A single intra-VTA microinjection of CNQX (1 μg, 10 min before light stimulation) significantly reduced the enhanced nAcc DA levels elicited by light stimulation (main effect group: F2,15=3.34,P=0.063; main effect time: F4,60=24.85,P<0.001; group × time interactions: F8,60=5.21,P=0.00006, two-way ANOVA). The 90-min time point samples from CNQX group were significantly different from the ones of ACSF group (*P<0.001, Bonferronipost hoctest, ACSF group: 290.0±58.7%; CNQX group: 129.0±10.3%), and although the AP5-treated group showed a slight decrease in evoked release of DA (90-min: 225.2±17.2%), it did not reach statistical significance. Figure 5: Light activation of VTA projections from DR VGluT3 neurons induces nAcc DA release mediated by VTA AMPA receptors. ( a ) Schematic representation of virus injection in DR of VGluT3::Cre mice, intra-VTA microinjection of AMPA receptor antagonist (CNQX), VTA light stimulation of DR-VGluT3 inputs, and microdialysis in nAcc. ( b ) VTA light activation of DR VGluT3 inputs induced nAcc DA release. Each point represents a 10-min dialysate sampling period (mean+s.e.m. percent of DA baseline); blue rectangles indicate the period of light stimulation. Light activation significantly enhanced nAcc DA levels in ChR2-eYFP mice ( n =6) but not in eYFP mice ( n =4) (main effect group: F 1,8 =96.91, P <0.001; main effect time: F 5,40 =42.17, P <0.001; group × time interactions: F 5,40 =40.38, P <0.001, two-way ANOVA). ( c ) nAcc DA release induced by VTA light activation of DR VGluT3 inputs is abolished by intra-VTA microinjection of CNQX but not AP5. Results were analysed separately for light activation only (10 to 70 min) and light activation following VTA microinjections of ACSF, CNQX or AP5 (80 to 120 min). Light activation significantly enhanced nAcc DA levels in all animals before VTA microinjections (main effect group: F 2,15 =0.37, P =0.70; main effect time: F 6,90 =22.36, P <0.001; group × time interactions: F 12,90 =0.15, P =1.00, two-way ANOVA). The 40-min time point samples were significantly different from all the other time point samples (# P <0.001, Bonferroni post hoc test, ACSF group: 297.7±79.7%, n =6; CNQX group: 292.5±69.3%, n =6; AP5 group: 250.9±29.2%, n =6). A single intra-VTA microinjection of CNQX (1 μg, 10 min before light stimulation) significantly reduced the enhanced nAcc DA levels elicited by light stimulation (main effect group: F 2,15 =3.34, P =0.063; main effect time: F 4,60 =24.85, P <0.001; group × time interactions: F 8,60 =5.21, P =0.00006, two-way ANOVA). The 90-min time point samples from CNQX group were significantly different from the ones of ACSF group (* P <0.001, Bonferroni post hoc test, ACSF group: 290.0±58.7%; CNQX group: 129.0±10.3%), and although the AP5-treated group showed a slight decrease in evoked release of DA (90-min: 225.2±17.2%), it did not reach statistical significance. Full size image Instrumental responding by VTA VGluT3-afferent activation By optogenetics, we determined whether activation of DR VGluT3 inputs to the VTA could establish and motivate instrumental responding. VGluT3-ChR2-eYFP or control (VGluT3-eYFP) mice were placed in chambers in which they were allowed to earn VTA optical stimulation by rotating response wheels; a quarter-turn of one of the wheels (‘active wheel’) resulted in the delivery of light into the VTA ( Fig. 6 and Supplementary Fig. 9 ). During the first period of six daily optical intracranial self-stimulation (oICSS) training sessions (30 min each), the right wheel was designated as the ‘active wheel’ ( Fig. 6a ). Each quarter-turn of the active wheel resulted in delivery of a 1 s train of 10-ms light pulses at a frequency of 20 Hz. The VGluT3-ChR2-eYFP mice rotated the ‘active wheel’ significantly more than the ‘inactive wheel’ from the first session on ( Supplementary Fig. 9a ), and significantly more than the VGluT3-eYFP mice turned either wheel ( P <0.001, three-way ANOVA, Fig. 6b ). To confirm that the frequency of wheel turning reflected a rewarding effect of the stimulation, we switched the active wheel for 4 days of reversal training following the first 6 days of training sessions. On the first reversal training day (RD1), ChR2-eYFP mice quickly changed preference to the new ‘active wheel’ ( Supplementary Fig. 9b ), on which they continued to respond for three subsequent reversal training sessions ( Fig. 6b ). When the mice were subsequently tested with different stimulation frequencies, it was found that stimulation at 1 Hz frequency was ineffective, but stimulations at 5, 10, 20 and 50 Hz were increasingly more effective ( Supplementary Fig. 9c ). The involvement of both glutamate AMPA and serotonin 5-HT2a and 5-HT2c receptors in the light-evoke instrumental responding were tested by intra-VTA microinjection of either the AMPA receptor antagonist (CNQX) or the 5-HT2a/5-HT2c receptors antagonist (ketanserin). While the number of wheel turns evoked by VTA VGluT3 light stimulation was significantly inhibited by the intra-VTA administration of CNQX ( P <0.05 versus ACSF group, two-way ANOVA, Supplementary Fig. 9d ), intra-VTA injection of ketanserin did not affect this behaviour. These findings indicate that instrumental responding evoked by VTA activation of the VGluT3 afferents is mainly mediated by AMPA receptors, and although some VGluT3 neurons synapsing on VTA DA neurons are also serotonergic, the release of serotonin from these VGluT3-serotonin neurons does not seem to have a role in this behaviour. 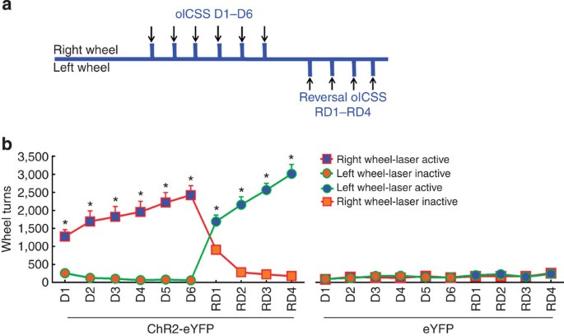Figure 6: Mice learn a wheel-turning response for light activation of VTA projections from DR VGluT3 neurons. (a) Diagram showing the timeline of the optical intracranial self-stimulation (oICSS) procedure: 6-day oICSS sessions (D1-D6, right wheel results in laser activation) and 4-day reversal oICSS sessions (RD1-RD4, left wheel results in laser activation). (b) Mean number of wheel turns in each session. VGluT3-ChR2-eYFP mice (n=9) rotated the ‘active’ response wheel significantly more than the ‘inactive’ wheel (*P<0.001, three-way ANOVA with Newman–Keulspost hoctest) and significantly more than VGluT3-eYFP mice (n=6) during the 6-day oICSS sessions (main effect group: F1,13=31.14,P<0.001, three-way ANOVA) and the 4-day reversal oICSS sessions (main effect group: F1,13=105.2,P<0.001, three-way ANOVA). Data are presented as mean+s.e.m. Figure 6: Mice learn a wheel-turning response for light activation of VTA projections from DR VGluT3 neurons. ( a ) Diagram showing the timeline of the optical intracranial self-stimulation (oICSS) procedure: 6-day oICSS sessions (D1-D6, right wheel results in laser activation) and 4-day reversal oICSS sessions (RD1-RD4, left wheel results in laser activation). ( b ) Mean number of wheel turns in each session. VGluT3-ChR2-eYFP mice ( n =9) rotated the ‘active’ response wheel significantly more than the ‘inactive’ wheel (* P <0.001, three-way ANOVA with Newman–Keuls post hoc test) and significantly more than VGluT3-eYFP mice ( n =6) during the 6-day oICSS sessions (main effect group: F 1,13 =31.14, P <0.001, three-way ANOVA) and the 4-day reversal oICSS sessions (main effect group: F 1,13 =105.2, P <0.001, three-way ANOVA). Data are presented as mean+s.e.m. Full size image VTA AMPA-mediated place preference by VGluT3-afferents Conditioned place preference was used to further characterize the rewarding properties of DR VGluT3 inputs to VTA. VGluT3-ChR2-eYFP and VGluT3-eYFP mice were tested in a three-chamber apparatus and given continuous trains of optical stimulation when they entered the laser-paired chamber ( Fig. 7 and Supplementary Fig. 10 ). The animals were able to terminate the stimulation by crossing back to the neutral chambers. VGluT3-eYFP mice spent similar time in both laser-paired and nonlaser-paired chambers, whereas VGluT3-ChR2-eYFP mice spent significantly more time in the laser-paired chambers ( P <0.05, three-way ANOVA, Fig. 7b ). When the VGluT3-ChR2-eYFP mice were subsequently tested in the absence of laser stimulation, they spent more time in the chamber where they had previously received the stimulation ( P <0.05, three-way ANOVA, Fig. 7b and Supplementary Fig. 10 ). Thus VGluT3-ChR2-eYFP mice not only earned the stimulation by entering the stimulation chamber when stimulation was available; they also acquired a preference for the stimulation-associated chamber as reflected by the time spent there on the subsequent day, when the stimulation was no longer available. 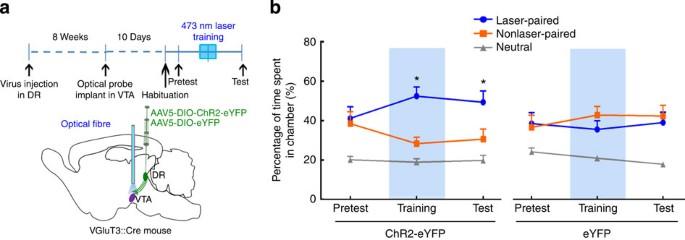Figure 7: Mice seek and return to the portion of the apparatus where they receive light activation of VTA projections from DR VGluT3 neurons. (a) Diagrams showing experimental timeline, virus injection in DR of VGluT3::Cre mice, and VTA light stimulation of DR VGluT3 inputs. (b) VGluT3-ChR2-eYFP mice (but not VGluT3-eYFP mice) sought out and spent more time in the chamber where VTA light stimulation was given during training. On the test day, VGluT3-ChR2-eYFP mice but not VGluT3-eYFP mice also returned to and spent more time in the chamber where light stimulation was given on the previous day (main effect group: F1,18=4.87,P<0.05, three-way ANOVA). Relative time spent in each chamber is represented as mean+s.e.m. (n=10 each group). Blue rectangles indicate light stimulation available in the laser-associated chamber. VGluT3-ChR2-eYFP mice showed preference for the laser-associated chamber on both training day and test day (*P<0.05, Newman–Keulspost hoctest). Figure 7: Mice seek and return to the portion of the apparatus where they receive light activation of VTA projections from DR VGluT3 neurons. ( a ) Diagrams showing experimental timeline, virus injection in DR of VGluT3::Cre mice, and VTA light stimulation of DR VGluT3 inputs. ( b ) VGluT3-ChR2-eYFP mice (but not VGluT3-eYFP mice) sought out and spent more time in the chamber where VTA light stimulation was given during training. On the test day, VGluT3-ChR2-eYFP mice but not VGluT3-eYFP mice also returned to and spent more time in the chamber where light stimulation was given on the previous day (main effect group: F 1,18 =4.87, P <0.05, three-way ANOVA). Relative time spent in each chamber is represented as mean+s.e.m. ( n =10 each group). Blue rectangles indicate light stimulation available in the laser-associated chamber. VGluT3-ChR2-eYFP mice showed preference for the laser-associated chamber on both training day and test day (* P <0.05, Newman–Keuls post hoc test). Full size image Finally, we evaluated the effects of intra-VTA injections of the AMPA receptor antagonist CNQX, and intra-nAcc injections of either the D1 receptor antagonist SCH23390 or the D2 receptor antagonist eticlopride on real-time place preference induced by VTA light activation of DR VGluT3 inputs. In these studies, CNQX (1 μg), ketanserin (1 μg), SCH23390 (0.1 μg) or eticlopride (1 μg) were each injected into the VTA or nAcc of different VGluT3-ChR2-eYFP mice 10 min before the laser-paired training ( Fig. 8a,c , and Supplementary Fig. 11 ). Mice that received a VTA or nAcc microinjection of ACSF showed preference to the laser-paired chamber on both laser training day ( P <0.05, three-way ANOVA) and test day ( P <0.05, three-way ANOVA, Fig. 8b,d ). In contrast, mice that received intra-VTA microinjection of CNQX or intra-nAcc microinjection of SCH23390 did not show preference for the laser-paired chamber on either laser training day or on test day. Intra-VTA microinjection of ketanserin or intra-nAcc microinjection of eticlopride did not affect the real-time place preference induced by VTA light activation of DR VGluT3 inputs ( Fig. 8b,d ). Together, these findings indicate that the DR VGluT3 inputs to the VTA mediate the development of place preference by releasing glutamate into the VTA, resulting in AMPA receptor activation on DA mesoaccumbens neurons that promotes D1 receptor activation within the nAcc via enhanced DA release. 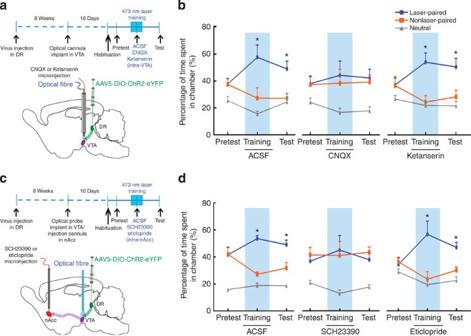Figure 8: VTA AMPA receptors mediate place preference evoked by light activation of projections from DR VGluT3 neurons. (a) Diagrams showing experimental timeline, virus injection in DR of VGluT3::Cre mice, VTA microinjection of CNQX or Ketanserin, and light stimulation of DR VGluT3 inputs. (b) Intra-VTA injection of CNQX (1 μg), but not Ketanserin (1 μg) blocked the development of real-time or conditioned preference for the side where light was delivered (main effect group: F2,17=2.52,P=0.115; group × time × chamber interaction: F8,68=3.3,P<0.005, three-way ANOVA). Relative time spent (mean+s.e.m.) in each chamber by mice. Mice received a single intra-VTA microinjection of ACSF (n=8), CNQX (n=6) or Ketanserin (n=6) 10 min before laser training. Intra-VTA ACSF or Ketanserin microinjected mice showed preference for the laser-associated chamber on training day and test day (*P<0.05, Newman–Keulspost hoctest). Intra-VTA CNQX microinjection blocked light-conditioned place preference. (c) Diagrams showing experimental timeline, virus injection in DR of VGluT3::Cre mice, nAcc microinjection of D1 receptor antagonist (SCH23390) or D2 receptor antagonist (Eticlopride), and light stimulation of DR VGluT3 inputs. (d) Intra-nAcc injection of SCH23390 (0.1 μg), but not eticlopride (1 μg) blocked the development of real time or conditioned preference for the side where light stimulation was delivered (main effect group: F2,16=2.45,P=0.118; group × time × chamber interaction: F8,64=3.1,P=0.005, three-way ANOVA). Relative time spent (mean+s.e.m.) in each chamber by mice. Mice received a single intra-nAcc microinjection of ACSF (n=7), SCH23390 (n=6), or eticlopride (n=6) 10 min before laser training. Intra-nAcc ACSF microinjected mice showed preference for the laser-associated chamber on training day and test day (*P<0.05, Newman–Keulspost hoctest). Intra-nAcc eticlopride microinjected mice showed preference to the laser-associated chamber on training day and test day (*P<0.05, Newman–Keulspost hoctest). Light-conditioned place preference was blocked by intra-nAcc microinjection of SCH23390. Figure 8: VTA AMPA receptors mediate place preference evoked by light activation of projections from DR VGluT3 neurons. ( a ) Diagrams showing experimental timeline, virus injection in DR of VGluT3::Cre mice, VTA microinjection of CNQX or Ketanserin, and light stimulation of DR VGluT3 inputs. ( b ) Intra-VTA injection of CNQX (1 μg), but not Ketanserin (1 μg) blocked the development of real-time or conditioned preference for the side where light was delivered (main effect group: F 2,17 =2.52, P =0.115; group × time × chamber interaction: F 8,68 =3.3, P <0.005, three-way ANOVA). Relative time spent (mean+s.e.m.) in each chamber by mice. Mice received a single intra-VTA microinjection of ACSF ( n =8), CNQX ( n =6) or Ketanserin ( n =6) 10 min before laser training. Intra-VTA ACSF or Ketanserin microinjected mice showed preference for the laser-associated chamber on training day and test day (* P <0.05, Newman–Keuls post hoc test). Intra-VTA CNQX microinjection blocked light-conditioned place preference. ( c ) Diagrams showing experimental timeline, virus injection in DR of VGluT3::Cre mice, nAcc microinjection of D1 receptor antagonist (SCH23390) or D2 receptor antagonist (Eticlopride), and light stimulation of DR VGluT3 inputs. ( d ) Intra-nAcc injection of SCH23390 (0.1 μg), but not eticlopride (1 μg) blocked the development of real time or conditioned preference for the side where light stimulation was delivered (main effect group: F 2,16 =2.45, P =0.118; group × time × chamber interaction: F 8,64 =3.1, P =0.005, three-way ANOVA). Relative time spent (mean+s.e.m.) in each chamber by mice. Mice received a single intra-nAcc microinjection of ACSF ( n =7), SCH23390 ( n =6), or eticlopride ( n =6) 10 min before laser training. Intra-nAcc ACSF microinjected mice showed preference for the laser-associated chamber on training day and test day (* P <0.05, Newman–Keuls post hoc test). Intra-nAcc eticlopride microinjected mice showed preference to the laser-associated chamber on training day and test day (* P <0.05, Newman–Keuls post hoc test). Light-conditioned place preference was blocked by intra-nAcc microinjection of SCH23390. Full size image Since the discovery of brain stimulation reward by Olds and Milner [17] , several experimental approaches have been used to characterize the underlying neural circuitry. Extensive mapping studies have identified dozens of brain sites where stimulation is rewarding, and paired-pulse parametric studies have linked different brain areas as part of the reward neural circuitry [18] , [19] , [20] . Connection between the DR and the VTA by common reward-associated fibres has been established by dual-electrode, paired-pulse stimulation experiments [3] , but these experiments did not reveal the origin or the target of the activated substrate. Electrical stimulation studies provide important information on the trajectory of fibres mediating reward functions, whereas optogenetic strategies have the capability of identifying the specific fibres involved in these functions. By combining optogenetics with anatomical, electrophysiological and behavioural approaches, we present evidence indicating that the DR provides a glutamatergic excitatory rewarding input to VTA dopamine neurons that project to the nAcc, our findings provide the first evidence of a reward-carrying input to the dopamine system in which the origin, neurotransmitter and synaptic termination of the input have been characterized. The DR has been classically recognized as a nucleus that contains an anatomically and functionally diverse population of serotonergic neurons [21] , [22] , [23] , [24] , many of which innervate brain areas involved in reward processing [7] , [8] , [9] , [10] , [25] . Given the broad distribution of serotonergic innervations on these brain areas, the role of serotonin on reward has been the subject of investigation for several decades. Although serotonin is generally considered to be antagonistic to reward function, the literature describing the role of serotonin on reward processing is complicated [26] , [27] , [28] , [29] . For example, serotonin-depleting drugs increase the response for brain stimulation reward [30] , [31] , [32] , consistent with an inhibitory role for serotonin on reward function. Similarly, local inhibition of serotonin neurons within the DR and median raphe facilitates brain stimulation reward [33] , and establishes conditioned place preference [34] . Place preference is also induced by other treatments thought to inhibit serotonergic function [35] , [36] . In contrast, others findings have suggested a role for DR serotonin in promoting reward [37] , [38] , including a recent optogenetic study demonstrating that photoactivation of DR neurons under the regulation of the Pet-1 promoter (selective promoter for brain serotonergic neurons) signals reward through serotonin and glutamate [38] . Although it has long been established that DR-serotonergic neurons densely innervate the VTA [9] , [10] , recent findings have shown that the VTA also receives innervation from DR-VGluT3 neurons [4] , [11] . Here we provide evidence indicating that in the rat and in the mouse the major input from the DR to VTA neurons is not from serotonergic neurons, but from VGluT3 neurons that establish synapses mostly on dopamine neuron. Midbrain dopamine neurons are not only responsive to rewards themselves; they are also responsive to reward-predictive stimuli [39] . Importantly, several in vivo electrophysiological studies in rodents and monkeys have shown that some DR neurons are excited by reward-predictive stimuli [40] , [41] , [42] , [43] , and that some DR Pet-1 neurons increase their firing activity during reward tasks [38] . Here we extend these findings by demonstrating that DR-VGluT3 neurons that synapse on mesoaccumbens DA neurons constitute a glutamatergic reward-carrying input to the dopamine system. While we found that activation of VGluT3 inputs from DR to VTA DA neurons is rewarding, we also noticed that the DR VGluT3 neurons innervate several brain areas previously shown to be involved in reward by electrical stimulation [2] , [3] , [17] . Thus we speculate that DR-VGluT3 neurons may mediate reward in other brain structures, and may be among the previously proposed ‘first stage’ neurons [17] in which direct activation may be responsible for the rewarding effect of stimulating the several brain sites that support self-stimulation [2] , [3] , [17] , and that may participate in diverse aspects of motivational brain function by releasing glutamate alone or together with serotonin. In this regard, we found that the rewarding effects of VGluT3 inputs to VTA DA neurons is mediated by VTA glutamatergic receptors without apparent contribution of VTA serotonergic receptors, which are expected to be affected by the co-release of serotonin from the dual VGluT3-serotonin terminals that also synapse on VTA neurons. However, we also found that many of the axon terminals synapsing on VTA neurons are from serotonin neurons lacking VGluT3, as such, they provide another pool of serotonin, the release of which may inhibit or synergize the excitatory actions resulting from the activation of VTA VGluT3 terminals. Although VTA receives inputs from several glutamatergic brain areas [4] , thus far, glutamatergic synapses on VTA DA neurons have been documented from neurons of the medial prefrontal cortex, mesopontine tegmentun nucleus, lateral habenula, periaqueductal grey [44] , [45] , [46] , [47] , [48] , [49] , and as shown in here by DR neurons. A recent study has demonstrated that different glutamatergic inputs to VTA can affect behaviour in unique ways, reward from the laterodorsal tegmental area or aversion from lateral habenula [50] . These observations indicate the importance of determining the contribution of selective inputs to VTA to better determine their role on behaviours associated with reward, aversion and motivation. In this regard, we found that even though the DR VGluT3 neurons preferentially synapse on DA neurons, they also synapse on VTA non-DAergic neurons, underscoring a complex participation of DR on VTA neuronal function. In summary, we found that although DR-serotonergic neurons provide a prominent input to the VTA, the DR glutamatergic neurons expressing VGluT3 are the major input from DR to VTA neurons in the rat and in the mouse. Within the VTA, these DR-VGluT3 neurons make asymmetric synapses mostly on dopamine neurons; some of these dopamine neurons specifically innervate the nucleus accumbens. Utilizing optogenetic approaches, we found that intra-VTA light stimulation of the VGluT3 fibres elicits AMPA-mediated excitatory currents on dopamine neurons that innervate the nucleus accumbens. Further, we report that such stimulation causes dopamine release in the nucleus accumbens, reinforces instrumental behaviour and establishes conditioned place preference. In conclusion, we report the discovery of a rewarding, excitatory synaptic input to the mesoaccumbens dopamine neurons by a glutamatergic projection arising from the DR-VGluT3 neurons. The discovery of this brain pathway opens new avenues to examine its participation in a variety of mental disorders related to motivation. Animals for anatomical studies Male Sprague–Dawley rats (9 weeks, n =4) or male wild-type C57Bl/6 mice (9 weeks, n =4) were anaesthetized with equithesin (3.3 ml kg −1 , intraperitoneal). The retrograde tracer Fluoro-Gold (FG; 1% in cacodylate buffer, pH 7.5, Fluorochrome) was delivered unilaterally into the VTA (coordinates in mm: for rat [57] AP −5.1, ML +0.5, DV −8.4; for mice [58] AP −3.3, ML +0.2, DV −4.3). FG was delivered iontophoretically through glass micropipette (20 μm) by applying 1 μA current in 5 s pulses at 10 s intervals for 20 min (rats) or 10 min (mice). The micropipette was left in place for an additional 10 min to prevent backflow. Male VGluT3::Cre mice [51] (breeding at least five generations, 8–10 weeks) were bred in the NIDA/IRP animal facility. Cre-inducible recombinant adeno-associated virus (AAV) vector was used to genetically target channelrhodopsin-2 (ChR2) expression to glutamate neurons in the DR of VGluT3::Cre mice. Mice were anesthetized with isoflurane (Butler Schein). Deeply anaesthetized mice were fixed in a stereotaxic apparatus (David Kopf Instruments), and 0.5 μl (0.1 μl min −1 ) AAV5-EF1a-DIO-hChR2(H134R)-mCherry or AAV5-EF1a-DIO-hChR2(H134R)-eYFP (3 × 10 12 genomes ml −1 , UNC Vector Core Facility) was injected using an NanoFil syringe (NANOFIL, WPI) into the DR (AP −4.3, ML ±0, DV −3.3). Eight weeks after viral injection into the DR, VGluT3-ChR2-mCherry mice ( n =4) were iontophoretically injected into the nAcc with 1% FG through glass micropipette by applying 3 μA current in 5 s pulses at 10 s intervals for 15 min (AP +1.4, ML ±0.8, DV −4.8/−4.2). One week following the FG injection, rats and VGluT3::Cre mice were anaesthetized and perfused transcardially with fixative solution (4% paraformaldehyde (PFA) for in situ hybridization-immunohistochemistry or 4% PFA in 0.1 M PB with 0.15% glutaraldehyde and 15% picric acid for fluorescent and electron microscopy]. For in situ hybridization-immunohistochemistry, coronal serial sections of 16 μm for DR and 30 μm for VTA were prepared. For fluorescent and electron microscopy, midbrain was cut into coronal serial sections (50 μm thick) with a vibratome (VT1000S, Leica). Rats were double housed, and all mice were housed in groups of up to four animals per cage in an animal room at 22 °C under a 12 h light/dark cycle (light on at 0700 hours), with ad libitum access to food and water. All animal procedures were approved by the NIDA Animal Care and Use Committee. Animals for functional studies For each optogenetic study, male VGluT3::Cre mice were injected with AAV5-EF1a-DIO-hChR2(H134R)-eYFP into the DR. Eight weeks after virus injection, the retrograde tracer Dil (D282, Life Technologies) was delivered into the nAcc (AP +1.4, ML ±0.8, DV −4.8/−4.2, 50 nl each site). Glass pipettes (20 μm) were filled with a 0.4% retrograde tracer DiI solution in ethanol. DiI was delivered by pressure through a glass micropipette attached to a Picospritzer III (Parker Hannifin Corporation). The micropipette was left for 10 min to prevent backflow. For microdialysis study, male C57Bl/6, VGluT3-ChR2-eYFP or VGluT3-eYFP mice were implanted with an unilateral microinjection guide cannula 1 mm above the VTA (AP −3.4, ML +0.3, DV −3.3) and a microdialysis guide cannula above the nAcc (AP +1.3, ML +0.6, DV −3.8). Mice were allowed to recover from surgery for 7 days before microdialysis. For oICSS and place preference experiments, VGluT3-ChR2-eYFP mice and VGluT3-eYFP mice were implanted with unilateral chronic optical fibres (200 μm diameter, BFL37-200, Thorlabs) directed above the VTA (AP −3.4, ML +0.3, DV −4.0) at 8 weeks after virus injection. For pharmacological studies, each mouse was implanted with a guide cannula (28-gauge, Plastics One) unilaterally 1 mm above the VTA (AP −3.4, ML +0.3, DV −3.3) or nAcc (AP +1.3, ML +1.3, DV −3.8, with 10° angle). Mice were allowed at least 10 days recovery before behavioural testing. Mice were assigned to the experimental groups according to the method of randomization. Rats or mice with retrograde tracer injection in anatomical or electrophysiological studies were excluded from data analysis if the injection sites were out of target. After microdialysis or behavioural test, brain sections from tested mice were examined. Mice with out-of-target cannula or probe implantation were excluded from the data analysis. Combination of in situ hybridization and immunolabeling Midbrain coronal free-floating sections were incubated for 2 h at 30 °C with rabbit anti-FG antibody (1:500, AB153, Millipore) and mouse anti-tryptophan hydroxylase (TPH, 1:500, T0678, Sigma) or guinea pig anti-VGluT3 antibody (1:1,000, AB5421, Millipore) in DEPC-treated phosphate buffer (PB) with 0.5% Triton X-100 supplemented with RNasin (40 U l −1 stock, 5 μl ml −1 of buffer, Promega). Sections were rinsed with 3 × 5 min DEPC-treated PB and incubated in biotinylated goat anti-rabbit antibody (1:200, Vector Laboratories) and fluorescein-conjugated donkey anti-mouse antibody (1:50, Jackson ImmunoResearch) for 1 h at 30 °C. Sections were rinsed with DEPC-treated PB and then transferred to 4% PFA. Sections were rinsed with DEPC-treated PB, incubated for 10 min in PB containing 0.5% Triton X-100, rinsed with PB, treated with 0.2 N HCl for 10 min, rinsed with PB and then acetylated in 0.25% acetic anhydride in 0.1 M triethanolamine, pH 8.0, for 10 min. Sections were rinsed with PB, and postfixed with 4% PFA for 10 min. Before hybridization and after a final rinse with PB, the sections were incubated in hybridization buffer for 2 h at 55 °C (50% formamide, 10% dextran sulfate, 5 × Denhardt’s solution, 0.62 M NaCl, 50 mM DTT, 10 mM EDTA, 20 mM PIPES, pH 6.8, 0.2% SDS, 250 μg ml −1 salmon sperm DNA, 250 g ml −1 tRNA). Sections were hybridized for 16 h at 55 °C in hybridization buffer containing [ 35 S]- and [ 33 P]-labelled single-stranded antisense VGluT3 (nucleotides 25–1,644; GenBank accession number: BC117229.1) probes at 10 7 c.p.m. ml −1 . Sections were treated with 4 μg ml −1 RNase A at 37 °C for 1 h and washed with 1 × saline-sodium citrate, 50% formamide at 55 °C for 1 h and with 0.1 × saline-sodium citrate at 68 °C for 1 h. Then sections were rinsed with PB and incubated for 1 h at room temperature in avidin-biotinylated horseradish peroxidase (1:200, ABC kit, Vector Laboratories). Sections were rinsed, and the peroxidase reaction was developed with 0.05% 3,3′-diaminobenzidine (DAB) and 0.03% H 2 O 2 . Sections were mounted on coated slides. Slides were dipped in Ilford K.5 nuclear tract emulsion (Polysciences, 1:1 dilution in double-distilled water) and exposed in the dark at 4 °C for 4 weeks before development. Data analysis of different phenotypes of FG-labelled neurons Sections were viewed, analysed and photographed with bright-field or epiluminescence microscopy using an Olympus BX51 microscope. Neurons were observed within each traced region at high power ( × 20 objective lenses) and marked electronically. Subdivisions of the DR were traced according to the rat brain atlas [57] . FG-VGluT3, FG-TPH, FG-VGluT3-TPH and FG-only labelled cells were analysed using epiluminescence to increase the contrast of silver grains [13] , [52] . For VGluT3 in situ hybridization procedures, FG fluorescent cells containing or lacking TPH fluorescent signal were photographed before processing for in situ hybridization. From radioactive in situ hybridization, a cell was considered to express mRNA when its soma contained concentric aggregates of silver grains above background level. A neuron was considered to express TPH-immunoreactivity when its soma was clearly seen as green fluorescence. A neuron was considered to express FG-immunoreactivity when its soma was clearly labelled as brown. FG-labelled cells (detected by fluorescence and brown DAB-label) expressing VGluT3 mRNA (detected by radioactive in situ hybridization) were counted separately. FG (brown DAB labelled) and radioactive in situ hybridization (silver grains) double-labelled material was analysed by the following procedure: (1) silver grains corresponding to VGluT3 mRNA expression were focused under epiluminescence microscopy, (2) the path of epiluminescence light was blocked without changing the focus and (3) bright-field light was used to determine whether a brown neuron, expressing FG in focus, contained the aggregates of silver grains seen under epiluminescence. The experiment was successfully repeated twice. Retrograde tract tracing cell counting was completed blindly by three different investigators. The data were collected from four rats (10–15 slides per rat) [13] , [52] . Fluorescence microscopy and three-dimensional analysis Free-floating coronal sections were incubated for 1 h in PB supplemented with 4% BSA and 0.3% Triton X-100. Sections were then incubated with cocktails of primary antibodies: mouse anti-TH antibody (1:1,000, MAB318, Millipore)+rabbit anti-FG antibody (1:2,000, AB153, Millipore); guinea pig anti-VGluT3 antibody (1:1,000, AB5421, Millipore)+rabbit anti-FG antibody (1:2,000, AB153, Millipore)+mouse anti-TPH (1:500, T0678, Sigma); guinea pig anti-VGluT3 antibody+rabbit anti-GluR1 antibody (1:200, GluR1C-Rb-Af692-1, Frontier Institute)+mouse anti-TH antibody; mouse anti-mCherry antibody (1:500, 632543, Clontech Laboratories)+rabbit anti-FG antibody+sheep anti-TH antibody (1:1,000, AB1542, Millipore); Cy5-Streptavidin (for biocytin detection; 43–8316, Life Technologies)+rabbit anti-TH antibody (1:1,000, AB152, Millipore)+mouse anti-GFP antibody (1:1,000, 632381, Clontech Laboratories), or mouse anti-mCherry antibody+guinea pig anti-VGluT3 antibody overnight at 4 °C. After rinsing 3 × 10 min in PB, sections were incubated in a cocktail of the corresponding fluorescence secondary antibodies (1:100, Alexa Fluor, Jackson Immunoresearch Laboratories) for 2 h at room temperature. After rinsing, the sections were mounted on slides. Fluorescent images were collected with an Olympus FV1000 Confocal System (Olympus). Images were taken sequentially with different lasers with × 100 oil immersion objectives and z axis stacks were collected at 0.2 μm. Amira microscopy software (Visualization Sciences Group, Burlington, MA) was used to analyze Z-stacks of confocal images from four rats or three VGluT3-ChR2-mCherry mice (64 × 64 × 10 μm for each image, four images from each animal) to obtain three-dimensional reconstruction of putative synapses [53] . This experiment was successfully repeated three times. Electron microscopy Vibratome tissue sections were rinsed with PB, incubated with 1% sodium borohydride in PB for 30 min to inactivate free aldehyde groups, rinsed in PB and then incubated with blocking solution (1% normal goat serum, 4% BSA in PB supplemented with 0.02% saponin) for 30 min. Sections were then incubated with primary antibodies as follows: guinea pig anti-VGluT3 (1:1,000)+mouse anti-TH antibodies (1:1,000), guinea pig anti-VGluT3+rabbit anti-GluR1 antibodies (1:200), or guinea pig anti-VGluT3+mouse anti-mCherry (1:1,000)+rabbit anti-FG antibodies (1:2,000). All primary antibodies were diluted in PB with 1% normal goat serum and incubations were for 24 h at 4 °C. Sections were rinsed and incubated overnight at 4 °C in the corresponding secondary antibodies: biotinylated goat anti-guinea pig antibody (for VGluT3 detection)+anti-mouse IgG fragment coupled to 1.4 nm gold (2001, Nanoprobes, 1:100 for TH detection), biotinylated goat anti-guinea pig antibody (for VGluT3 detection)+anti-rabbit IgG coupled to 1.4 nm gold (2003, Nanoprobes, 1:100 for GluR1 detection), biotinylated goat anti-mouse antibody (for mCherry detection)+anti-guinea pig IgG Fab’ fragment coupled to 1.4 nm gold (1:100 for VGluT3 detection)+anti-rabbit IgG coupled to 1.4 nm gold (1:100 for FG detection). Sections were rinsed in PB, and then in double-distilled water, followed by silver enhancement of the gold particles with the Nanoprobe Silver Kit (2012, Nanoprobes) for 7 min at room temperature. Next, sections were incubated in avidin-biotinylated horseradish peroxidase complex (1:100, ABC, Vector Laboratories) in PB for 2 h at room temperature and washed in PB. Peroxidase activity was detected by placing the sections in a solution containing 0.025% DAB and 0.003% H 2 O 2 in PB for 5–10 min. Sections were rinsed with PB and fixed with 0.5% osmium tetroxide in PBS for 25 min, washed in PBS followed by double-distilled water and then contrasted in freshly prepared 1% uranyl acetate for 35 min. Sections were dehydrated through a series of graded alcohols and with propylene oxide. Afterwards, they were flat embedded in Durcupan ACM epoxy resin (14040, Electron Microscopy Sciences). Resin-embedded sections were polymerized at 60 °C for 2 days. Sections of 65 nm were cut from the outer surface of the tissue with an ultramicrotome UC7 (Leica Microsystems) using a diamond knife (Diatome). The sections were collected on formvar-coated single slot grids and counterstained with Reynolds lead citrate. Sections were examined and photographed using a Tecnai G 2 12 transmission electron microscope (Fei Company) equipped with a digital micrograph 3.4 camera (Gatan) [54] . Ultrastructural analysis Serial thin sections of rat VTA (bregma −5.02 to −6.36 mm; ref. 57 ) and mouse VTA (bregma −2.92 to −3.88 mm; ref. 58 ) were used in this study. Synaptic contacts were classified according to their morphology, immunolabel and photographed at a magnification of × 6,800–13,000. Large and medium sized dendrites were identified by the presence of endoplasmic reticulum, mitochondria and microtubules. Dendritic spines were identified by the absence of mitochondria. Axon terminals were characterized by the presence of synaptic vesicles and mitochondria, whereas axon pre-terminals and unmyelinated axons are smaller in diameter and occasionally contained a small number of synaptic vesicles. Serial sections were obtained to determine the type of synapse. Type 1 synapses are referred to as symmetric synapses and have thin postsynaptic densities; whereas type 2 synapses, referred to as asymmetric synapses, were characterized by the presence of postsynaptic densities with thickness >40 nm (ref. 56 ). In the serial sections, a terminal containing >10 immunogold particles was considered an immunopositive terminal. Pictures were adjusted to match contrast and brightness by using Adobe Photoshop (Adobe Systems). The data were collected from four rats and three VGluT3::Cre mice [54] . This experiment was successfully repeated three times. Both quantification of electron microscopic and confocal analysis were done blindly. Slice preparation and optogenetic electrophysiology Electrophysiological data were obtained from six mice to minimize intra-subject variability. One week after DiI injection, VGluT3-ChR2-eYFP mice were anaesthetized with isoflurane and decapitated. Brains were removed and placed in ice-cold cutting buffer consisting of (in mM) 93 NMDG, 2.5 KCl, 0.5 CaCl 2 , 10 MgSO 4 , 25 glucose, 20 HEPES, 30 NaHCO 3 , 1.2 NaH 2 PO 4 , 5 sodium ascorbate, 3 sodium pyruvate, and 2 thiourea (pH 7.2–7.3; 300–310 mOsm). Dissected brains were cut into 220 μm horizontal sections on a vibratome (VT1000S; Leica) in ice-cold cutting buffer. Sections were transferred to 34 °C cutting buffer for 12~15 min, and then transferred to room temperature oxygenated (95% O 2 /5% CO 2 ) ACSF containing (in mM)126 NaCl, 3 KCl, 2.4 CaCl 2 , 1.5 MgCl 2 , 11 glucose, 26 NaHCO 3 , 1.2 NaH 2 PO 4 . During recordings, slices were maintained at ~32 °C, and picrotoxin (100 μM) was included in the perfusion ACSF to block GABA A receptors. Whole-cell voltage clamp recordings on DiI positive neurons in the VTA were obtained under visual guidance using an upright microscope (Olympus BX51) equipped with differential interference contrast-infrared (DIC-IR) illumination and fluorescence. Recordings were obtained using 3–6 MΩ resistance pipettes backfilled with internal solution containing (in mM)140 potassium gluconate, 2 NaCl, 1.5 MgCl 2 , 10 HEPES, 4 Mg-ATP, 0.3 Na 2 -GTP, 10 Tris-phosphocreatine, 0.1 EGTA and 0.2% biocytin (pH 7.2; 287 mOsm). Currents were measured using an Axoclamp 200B amplifier (2 kHz low-pass Bessel filter) and acquired to PC using a National Instruments data acquisition board (10 kHz digitization) and Windows-based software (WinLTP 2.01). Neurons were voltage clamped at −70 mV. An optical fibre (200 μm) coupled to a 473 nm laser was placed within the bath and focused near the site of recording, and was used to deliver 5 ms, 5 mW optical stimulation in paired pulses or a train of 10 pulses at 5–50 Hz. Experiments indicated that these conditions were saturating for light-evoked EPSCs (data not shown). Series resistance (5–20 MΩ) was monitored online with a 10 mV hyperpolarizing step (100 ms) following each stimulus. Sweeps were collected every 30 s. AMPA currents were blocked by bath application of 10 μM DNQX. To quantify the effect of drugs, sweeps were averaged for the last 2 min of the pre- and post-drug phases of the experiment. Before drug application, current clamp recordings were also performed to determine if glutamate from VGluT3 terminals could promote neuronal firing. In these recordings, a small amount of holding current was applied to maintain the membrane potential between −55 and −60 mV. Because we were only interested in sampling from a known population of cells (DiI-labelled), we confined our statistical analyses to these cells. To verify the monosynaptic connection between DR VGluT3 axons and VTA DA neurons, TTX (500 nM) and 4-aminopyridine (200 μM) were bath applied in succession. Latency of the optical-evoked EPSCs was defined as the interval between the onset of the laser pulse and the time point at which 10% of the peak amplitude was achieved. Latency and jitter (standard deviation of latency) was calculated from 20 successive recordings for each VTA neuron. In vivo microdialysis and quantification of DA A microdialysis probe (0.24 × 1 mm, CMA7, CMA Microdialysis) was inserted into the guide cannula implanted in the nAcc of VGluT3-ChR2-eYFP ( n =6) or VGluT3-eYFP ( n =4) mice in the evening before testing. The inlet tubing of the probe was connected to a microinfusion pump (CMA 100) via a fiber-optic and liquid rotary joint (Doric Lenses), and animals were placed into chambers (20 × 30 × 35 cm). Probes were perfused with ACSF (in mM: 140 NaCl, 2.7 KCl, 1.2 MgCl 2 , 1.4 CaCl 2 , 5 glucose, adjusted to pH 7.3–7.4 using NaOH) overnight at a flow rate of 0.2 μl min −1 . The following day, an optical fibre was inserted into the VTA through the guide cannula, and perfusate was replaced with fresh ACSF at the flow rate of 2.4 μl min −1 . Following a 3-h equilibration period, microdialysis samples were collected every 10 min into 5 μl 0.1 M perchloric acid to prevent DA degradation. Three 10 min samples were collected to determine the baseline of DA release in nAcc. Optical stimulation was delivered via optical fibre into the VTA for 10 min (473 nm, 1 mW, 10 ms, 20 Hz, 3 s on/off). To test the involvement of VTA glutamate AMPA or NMDA receptors, after the optical stimulation, three consecutive samples were collected before microinjection with ACSF, CNQX (1 μg), or AP5 (1 μg) ( n =6 each group) into the VTA. One 10 min sample was collected after the microinjection followed by another 10 min optical stimulation in the VTA. Three more consecutive samples were collected after the optical stimulation. DA concentration was measured by reverse-phase HPLC with electrochemical detection. Dialysate was injected into an Eicom HTEC-500 HPLC system containing a HPLC column (PP-ODS2, 4.6 × 30 mm), a HTEC-500 pump, and an integrated amperometric detector. The mobile phase consisted of (in mM) 100 NaH 2 PO 4 , 1.3 EDTA, 2.0 decane-1-sulfonate, 0.5% methanol, pH 5.4. Applied potential was set at +400 mV versus Ag/AgCl. Concentration of dialysate DA levels were estimated using calibration curves obtained from external standards. Detection limit of DA using these conditions was approximately 50 pM. Behavioural studies The glutamate AMPA receptor antagonist CNQX (#C239), NMDA receptor antagonist AP5 (#A5282), serotonin 5-HT2a and 5-HT2c receptor antagonist ketanserin (#S006), dopamine D1 receptor antagonist SCH23390 (#D054) and D2 receptor antagonist eticlopride (#E101) were obtained from Sigma and dissolved in ACSF. Volume of 0.2 μl was microinjected in behavioural studies. A three-chamber conditioned place preference apparatus was used for the real-time place preference test (Anymaze, Stoelting), which consisted of two chambers (20 × 18 × 35 cm) with distinct walls patterns and floors, and a connecting chamber (20 × 10 × 35 cm). The animal’s position was monitored via a CCD camera. For oICSS a sound-attenuated operant chamber was used. An optical encoder was attached next to the response wheel and recorded each 90° turn of the wheel (Med Associates). Each chamber was connected to a computer interface running software (MED-PC for Windows) that recorded wheel turns and issued the laser stimulation. VGluT3-ChR2-eYFP ( n =9) and VGluT3-eYFP ( n =6) mice each with a unilateral chronic optical fibre were used for oICSS. After 10 days recovery, mice were placed into the operant chambers featured with two wheels (right wheel and left wheel). They were trained on a fixed ratio (FR1) reinforcement schedule; each time the mouse rotated the active response wheel by 90°, the computer delivered a 1-s 20 Hz optical pulse train of light stimulation (473 nm, 20 mW, 5 ms duration). Each daily training session lasted 30 min. For six oICSS training sessions, the right wheel was designated as the ‘active wheel’: quarter turns on this wheel caused delivery of light stimulation. Reversal training was given for the next four training days; here the left wheel became the ‘active wheel’. We recorded both active and inactive wheel turns during the 10 days. One week after oICSS training at frequency of 20 Hz, the VGluT3-ChR2-eYFP mice ( n =8) were retested in 30-min daily sessions at five different stimulation frequencies (1, 5, 10, 20 and 50 Hz), given in counterbalanced order. Four mice received five different stimulation frequencies in the ascending order and the other four received stimulation frequencies in the descending order. To test the participation of VTA glutamate AMPA receptors or serotonin receptors in instrumental responding, VGluT3-ChR2-eYFP mice that were oICSS-trained for 6 days received an intra-VTA microinjection of ACSF, CNQX (AMPA receptor antagonist, 1 μg) or ketanserin (5-HT2a/5-HT2c receptor antagonist, 1 μg, ref. 55 ) 10 min before being placed in the place preference apparatus. The active wheel rotation resulted in 20 Hz light stimulation, and both active and inactive wheel turns were recorded in the 30-min session. VGluT3-ChR2-eYFP and VGluT3-eYFP mice were used for real-time place preference. Here, on each of the four days, mice were connected to an optical fibre and allowed to access the three chambers of the apparatus freely. On habituation day and pretest day, mice were connected to an optical fibre with no laser (15-min session). Mice showing side preference were excluded. On laser training day (30-min session), one chamber was randomly assigned as the stimulation chamber (counterbalanced across all mice). Whenever the mouse was within the stimulation chamber the laser was on (473 nm, 1 mW, 10 ms duration at 20 Hz, Fig. 7a ). On test day (15-min session), the mice were allowed to freely explore the three chambers without optical stimulation. To test whether the real-time place preference was affected by the laser intensity, while maintaining the frequency (20 Hz) and duration of the pulses (10 ms duration) laser stimulation was delivered in the descending order of intensity (1, 5 and 20 mW) in the same group of animals. Each animal was run throughout the three-day place preference procedure for each intensity, but allowing a period of 10 days between each three-day procedure. To test the participation of VTA glutamate AMPA receptors and nAcc dopamine D1/D2 receptors in the real-time place preference, we administered microinjections of ACSF, CNQX (1 μg) or ketanserin (1 μg) in the VTA, and ACSF, SCH23390 (D1 receptor antagonist, 0.1 μg) or eticlopride (D2 receptor antagonist, 1 μg) in the nAcc. VGluT3-ChR2-eYFP mice were implanted with a guide cannula above the VTA 10 days prior to behavioural testing (training timeline shown in Fig. 8a,c ). A microneedle was inserted 1 mm below the tip of the guide cannula. Each infusion was done with a microprocessor-controlled infusion pump and lasted 1 min. The microneedle was removed 1 min after infusion, and real-time place preference test was performed 10 min after infusion. The mice were given optical stimulation (473 nm, 1 mW, 10 ms duration at 20 Hz) on laser training day. Locomotor activity was recorded during the whole behavioural test. Statistics analysis All the statistical analyses applied in anatomy studies were performed with GraphPad Prism 5. In electrophysiological studies, we performed unpaired t -test, paired t -test, a Pearson’s correlation or two-way ANOVA to analyze the data when applicable. We performed two or three-way ANOVA to analyse the microdialysis and behavioural data when applicable. ANOVA was followed by a post hoc Bonferroni or Newman–Keuls test for multiple comparisons. Statistical analyses were performed with STATISTICA 9. P <0.05 was considered significant. How to cite this article : Qi, J. et al. A glutamatergic reward input from the dorsal raphe to ventral tegmental area dopamine neurons. Nat. Commun. 5:5390 doi: 10.1038/ncomms6390 (2014).